Cdo suppresses canonical Wnt signalling via interaction with Lrp6 thereby promoting neuronal differentiation Canonical Wnt signalling regulates expansion of neural progenitors and functions as a dorsalizing signal in the developing forebrain. In contrast, the multifunctional co-receptor Cdo promotes neuronal differentiation and is important for the function of the ventralizing signal, Shh. Here we show that Cdo negatively regulates Wnt signalling during neurogenesis. Wnt signalling is enhanced in Cdo-deficient cells, leading to impaired neuronal differentiation. The ectodomains of Cdo and Lrp6 interact via the Ig2 repeat of Cdo and the LDLR repeats of Lrp6, and the Cdo Ig2 repeat is necessary for Cdo-dependent Wnt inhibition. Furthermore, the Cdo-deficient dorsal forebrain displays stronger Wnt signalling activity, increased cell proliferation and enhanced expression of the dorsal markers and Wnt targets, Pax6, Gli3, Axin2. Therefore, in addition to promoting ventral central nervous system cell fates with Shh, Cdo promotes neuronal differentiation by suppression of Wnt signalling and provides a direct link between two major dorsoventral morphogenetic signalling pathways. Development of the central nervous system (CNS) is a multistep process that requires coordinated events, including cell fate specification, proliferation of neural progenitors (NPCs) and terminal differentiation to produce adequate numbers of mature neurons. The precise control of these events spatially as well as temporally is critical to ensure normal brain development. Several classes of secreted factors and signalling pathways are implicated in the regulation of neurogenesis and brain development. Among these, Shh and Wnt signalling are thought to play important roles in CNS development [1] , [2] . Wnts are secreted glycoproteins that trigger intracellular signalling pathways known as canonical and noncanonical Wnt signalling. In canonical Wnt signalling (simply referred as Wnt signalling), Wnts, such as Wnt1, 3 and 3a, bind to Frizzled receptors and low-density lipoprotein receptor-related protein (Lrp) 5 or 6 co-receptor complexes, leading to stabilization and translocation of β-catenin into the nucleus, followed by transcription activation of target genes [3] . The targeted mutagenesis of Wnts and downstream components of Wnt signalling suggested the functional importance of Wnt signalling in various aspects of CNS development [4] . However, the molecular mechanisms of Wnt signalling in neurogenesis appear to be complex but distinct depending on the temporal and spatial context during CNS development. In general, Wnt signalling is believed to promote proliferation of NPCs, most likely via induction of pro-proliferative target gene expression such as Cyclin D1 or c-Myc [5] , [6] . Inhibition of Wnt signalling by overexpression of a dominant negative form of activator, an inhibitory component Axin or the brain-specific ablation of β-catenin has been shown to promote neuronal differentiation, both in developing embryos as well as in embryonic stem cells [7] , [8] , [9] . In addition, inhibition of Wnt signalling by deletion of Wnt1 or Lrp6 in embryonic stem cells enhanced dopaminergic neuronal differentiation [10] . Conversely, the expression of an active form of β-catenin leads to inhibition of neural differentiation and an expansion of undifferentiated progenitors ultimately resulting in brain enlargement [11] . Together, these reports indicate that Wnt signalling controls expansion of NPCs during brain development. Given the diverse roles of Wnt signalling in neurogenesis, a tight control of this signalling will be critical; however, the precise regulatory mechanism by which Wnt signalling regulates neurogenesis is still largely unclear. The multifunctional co-receptor Cdo is a member of the immunoglobulin (Ig) superfamily and is highly expressed in the CNS and skeletal muscles during embryogenesis. Consistent with its expression pattern, Cdo plays important roles in myogenesis and neurogenesis [12] , [13] . In myoblasts, Cdo promotes differentiation as a component of multiprotein complexes that include the cell adhesion molecules N-cadherin and the closely related proteins Boc and Neogenin [14] , [15] , [16] . Among multiple downstream signalling events, p38MAPK positively regulates the activity of myogenic bHLH factors, such as MyoD, via phosphorylation of the ubiquitously expressed E-protein-binding partners of the myogenic as well as neural bHLH factors [17] , [18] . Consistently, Cdo also promotes neuronal differentiation by stimulation of transcriptional activity of Neurogenin1 in P19 embryonal carcinoma cells [19] . Furthermore, Cdo is required for neurogenesis in vivo , as suggested by decreased proliferation and neuronal differentiation of cortical NPCs isolated from Cdo-deficient embryos resulting in reduced cortical thickness and multiple defects in brain development of Cdo-mutant mice, including holoprosencephaly and hydrocephalus [13] , [20] . In early forebrain development, Wnt signalling regulates the expansion and specification of the dorsal neuroepithelial cells and is involved in patterning of the dorsal forebrain, while Shh signalling from the floor plate counteracts Wnt signalling thereby controlling the ventral cell fates [21] , [22] . Cdo is implicated in early forebrain development as a co-receptor of Shh signalling to activate the downstream signalling. Cdo-deficient mice exhibit defects in ventral neural cell fate specification and ventral forebrain development in correlation with decreased Shh signalling [20] , [21] , [22] , [23] , [24] . At the early embryonic stage before embryonic day 12 (E12), the transient expression of Cdo in the prechordal mesoderm or notochord appears to be critical for the full activation of Shh signalling to specify the ventral cell fates. However, the highest expression of Cdo is observed in the dorsal forebrain where Wnt signalling is high and Shh signalling is yet to occur [23] , suggesting that Cdo may have a distinct function in the dorsal forebrain, independent of Shh. In this study, we investigate a cross-regulation between Cdo and Wnt signalling in neurogenesis and in the developing forebrain. Our study suggests that Cdo induces neuronal differentiation through suppression of Wnt signalling by multiple mechanisms including direct Lrp6 binding and Wnt expression. Cdo deficiency caused an increase in Wnt signalling To investigate the interaction between Cdo and Wnt signalling in neurogenesis, we first assessed Wnt signalling activation during neuronal differentiation of P19 cells. To do so, P19 cells were induced to differentiate by treatment with 0.5 μM retinoic acid (RA) for 2 days in insulin/transferin/selenium medium (ITS) and further cultured without RA in ITS medium. Cells were harvested at proliferating in serum-containing medium (G) or various differentiation time points and total RNAs were purified, followed by semiquantitative reverse transcriptase–PCR (RT–PCR) analysis for expression of canonical Wnts, Wnt1 and Wnt3, and a pan-neuronal marker β-tubulin III for neuronal differentiation ( Supplementary Fig. 1a ). Wnt1 and Wnt3 transcripts were dramatically induced upon RA treatment when P19 EC cells were induced to differentiate into neuronal progenitors. Furthermore, the activation of β-catenin was assessed by nuclear fractionation and immunoblotting. The level of an active, unphosphorylated form of β-catenin (β-catenin*) was high in cells at the proliferating pluripotent stage (G) and transiently further increased on day 1 of RA treatment (RA1), while total β-catenin levels stayed relatively constant ( Supplementary Fig. 1b ). Consistently, the level of nuclear β-catenin accumulation was highest at RA1 ( Supplementary Fig. 1c ). As previously shown, Cdo was strongly induced upon RA treatment and returned to the basal level on day 1 without RA (ITS1) when the cells are expressing a pan-neuronal marker β-tubulin III. In addition, the expression of Wnt co-receptors, Lrp5 and Lrp6, was analysed in P19 cells ( Supplementary Fig. 1d ). Lrp5 was expressed in proliferating P19 cells until RA1 but downregulated in differentiating cells, while Lrp6 was strongly induced upon RA treatment similarly to Cdo. Taken together, the activation of Wnt signalling and the expression of Wnt signalling components, including Wnts and Lrp6, are strongly induced at the early specification stage of neurogenesis. Since both Wnt signalling and Cdo expression are increased upon induction of neurogenesis, we next examined the effect of Cdo-overexpression or knockdown on Wnt signalling and neuronal differentiation of P19 cells and C17.2 NPCs. P19 cells transfected with pcDNA (−) or Cdo (+) expression vectors were assessed for the activation of Wnt signalling at RA1 ( Fig. 1a ). The level of β-catenin* and an active, phosphorylated form of Lrp6 (pLrp6) decreased greatly in Cdo-overexpressing cells, compared with control cells. In addition, total β-catenin, Cyclin D1 and Lrp6 proteins were also reduced in these cells. Consistently, Cdo-overexpression in C17.2 cells had similar effects on Wnt signalling and resulted in strongly increased β-tubulin III expression ( Supplementary Fig. 2a ). Furthermore, the quantitative RT–PCR (qPCR) analysis with RNAs isolated from pcDNA or Cdo-transfected P19 cells at G or RA1 showed decreased expression of a Wnt target gene Axin2 in both conditions, while Wnt3 transcription only decreased at RA1 ( Fig. 1b ). To further analyse the β-catenin transactivation activity, P19 cells were co-transfected with the control or two varying amounts (0.5 and 1 μg) of Cdo expression vectors along with the Top-flash reporter. The higher amount of Cdo resulted in 50% of the Top-flash reporter activity relative to the control ( Fig. 1c ). Conversely, Cdo-depletion in P19 cells by Cdo-short hairpin RNA (shRNA) caused strongly increased levels of β-catenin*, total β-catenin, Cyclin D1 and pLrp6 proteins, while Lrp6 levels stayed unaltered, compared with control-shRNA cells ( Fig. 1d ). In addition, total RNA was harvested from these cells at G or RA1, followed by qPCR analysis ( Fig. 1e ). Cdo-depleted cells exhibited an increase in Wnt3 and Axin2 expression in both culture conditions. Similarly to P19 cells, Cdo-depletion in C17.2 cells enhanced Wnt signalling, accompanied by increased Cyclin D1 proteins. In agreement with our previous data [20] , Cdo-depleted cells expressed less β-tubulin III compared with control cells, suggestive of impaired neuronal differentiation ( Supplementary Fig. 2b ). In addition, the nuclear β-catenin levels were substantially increased in Cdo-depleted P19 cells, while the cytoplasmic β-catenin was relatively constant ( Fig. 1f ). We further analysed the effect of Cdo deficiency on Wnt signalling with Cdo +/+ and Cdo −/− NPCs isolated from embryonic forebrains on E12. Proteins and RNAs were harvested from NPCs induced to differentiate by bFGF removal for 2 (D2) to 3 days followed by immunoblotting and qPCR analysis. The level of pLrp6 was roughly 1.5-fold higher in Cdo −/− NPCs, compared with Cdo +/+ cells, while total Lrp6 proteins were slightly decreased ( Fig. 1g and Supplementary Note 1 ). Furthermore, Wnt3a and Axin2 mRNA expression levels were substantially enhanced in Cdo −/− NPCs, compared with Cdo +/+ cells ( Fig. 1h ). In addition, Cdo +/+ and Cdo −/− NPCs were treated with either bovine serum albumin (BSA) or 20 ng ml −1 Wnt3a and analysed for the nuclear accumulation of β-catenin by immunostaining. Cdo −/− NPCs exhibited more cells with nuclear β-catenin accumulation, compared with Cdo +/+ cells in both conditions ( Fig. 1i,j ). Since Wnt signalling activities and the expression of signalling components including Lrp6 fluctuated during neuronal differentiation of P19 cells, we have further assessed Wnt signalling in Cdo +/+ and Cdo −/− mouse embryonic fibroblasts (MEFs). Similar effects of Cdo deficiency on Wnt signalling were observed in Cdo +/+ or Cdo −/− MEFs. Consistently, the levels of pLrp6, β-catenin* and Cyclin D1 were significantly increased in Cdo −/− MEFs relative to Cdo +/+ cells ( Supplementary Fig. 2c ). The cellular fractionation of MEFs showed similar results as observed in P19 cells ( Supplementary Fig. 2d ). The Wnt-reporter activity was increased about three-fold in Cdo −/− cells compared with that of Cdo +/+ cells, which was set to 1 ( Supplementary Fig. 2e ). As a positive control, Cdo +/+ MEFs were treated with 5 mM LiCl for 24 h and the luciferase activity was increased ~5.8-fold. These data suggest that Cdo deficiency enhances Wnt signalling in various cell types, including MEFs and NPCs. 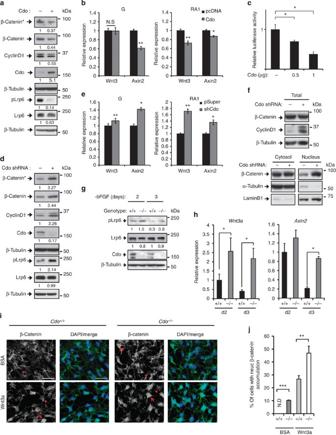Figure 1: Cdo deficiency enhanced Wnt signalling. (a) Immunoblot analysis of P19/pcDNA or P19/Cdo cell lysates at RA1. The quantification of normalized signal intensities relative to β-tubulin is shown below each lane and the signals in the control lane are set to 1. (b) qPCR of RNAs isolated from P19/pcDNA or P19/Cdo cells at G or RA1. (c) Luciferase assays of P19 cells expressing the control or two varying amounts (0.5 and 1 μg) of Cdo. The results were plotted as relative luciferase activities. (d) Immunoblotting of P19/control or P19/Cdo-shRNA cells at RA1. The quantification of the normalized signal intensity is shown below each lane. (e) qPCR of RNAs isolated from P19/control or P19/Cdo-shRNA cells at G or RA1. (f) Cellular fractionation and immunoblotting of P19/control or P19/Cdo-shRNA cells at RA1. (g) Immunoblot analysis with extracts ofCdo+/+andCdo−/−NPCs at the indicated differentiation days. (h) qPCR with RNAs isolated fromCdo+/+andCdo−/−NPCs at the indicated differentiation time points. (i) Confocal microscopy ofCdo+/+andCdo−/−NPCs treated with BSA or 20 ng per ml Wnt3a for 24 h on differentiation day 2, followed by immunostaining for β-catenin. Size bar=20 μm. (j) Quantification of the nuclear β-catenin accumulation from data shown ini. For example, cells marked with a red arrow iniare counted as positive for nuclear β-catenin accumulation, while cells marked with an arrowhead are counted as negative. The mean values of at least 10 fields. This experiment was performed three times with three batches of NPCs. Data are presented in this figure as mean±s.d. All experiments were repeated at least three times with similar results, unless differently stated. *P<0.05, **P<0.01, ***P<0.005. Statistical significance was tested by a Student’st-test. Figure 1: Cdo deficiency enhanced Wnt signalling. ( a ) Immunoblot analysis of P19/pcDNA or P19/Cdo cell lysates at RA1. The quantification of normalized signal intensities relative to β-tubulin is shown below each lane and the signals in the control lane are set to 1. ( b ) qPCR of RNAs isolated from P19/pcDNA or P19/Cdo cells at G or RA1. ( c ) Luciferase assays of P19 cells expressing the control or two varying amounts (0.5 and 1 μg) of Cdo. The results were plotted as relative luciferase activities. ( d ) Immunoblotting of P19/control or P19/Cdo-shRNA cells at RA1. The quantification of the normalized signal intensity is shown below each lane. ( e ) qPCR of RNAs isolated from P19/control or P19/Cdo-shRNA cells at G or RA1. ( f ) Cellular fractionation and immunoblotting of P19/control or P19/Cdo-shRNA cells at RA1. ( g ) Immunoblot analysis with extracts of Cdo +/+ and Cdo −/− NPCs at the indicated differentiation days. ( h ) qPCR with RNAs isolated from Cdo +/+ and Cdo −/− NPCs at the indicated differentiation time points. ( i ) Confocal microscopy of Cdo +/+ and Cdo −/− NPCs treated with BSA or 20 ng per ml Wnt3a for 24 h on differentiation day 2, followed by immunostaining for β-catenin. Size bar=20 μm. ( j ) Quantification of the nuclear β-catenin accumulation from data shown in i . For example, cells marked with a red arrow in i are counted as positive for nuclear β-catenin accumulation, while cells marked with an arrowhead are counted as negative. The mean values of at least 10 fields. This experiment was performed three times with three batches of NPCs. Data are presented in this figure as mean±s.d. All experiments were repeated at least three times with similar results, unless differently stated. * P <0.05, ** P <0.01, *** P <0.005. Statistical significance was tested by a Student’s t -test. Full size image Wnt inhibition restored neurogenesis in Cdo-depleted cells Next, P19 cells transfected with expression vectors for the control or Cdo-shRNA with Top-flash and β-galactosidase were treated with either dimethylsuphoxide (DMSO) or XAV939 (4 μM) in differentiation medium for 24 h followed by the luciferase assay. XAV939-treated control cells showed a reduction of Wnt-reporter activities to roughly 50% of the DMSO-treated control. In addition, the reporter activity was increased ~2.5-fold in Cdo-depleted cells and this increase was suppressed by the XAV939 treatment nearly to the levels of the control cells ( Fig. 2a ). P19/control or P19/Cdo shRNA cells were treated with DMSO or XAV939 in the differentiation medium for 72 h followed by immunostaining. To quantify, clusters containing the indicated numbers of β-tubulin III-positive cells were counted and plotted as percentile. XAV939-treated control cells displayed a modest increase in β-tubulin III-positive cells, compared with the control-treated cells. Furthermore, Cdo-depleted P19 cells treated with DMSO exhibited a significant reduction in β-tubulin III-positive cells, while XAV939 treatment restored neuronal differentiation of these cells nearly to the control level ( Fig. 2b,c ). In addition, XAV939-treated control cells showed increased β-tubulin III expression, compared with DMSO-treated cells ( Fig. 2d ). Furthermore, Cdo +/+ and Cdo −/− NPCs treated with DMSO or XAV939 for 1 day at D2 were examined with qPCR analysis. Axin2 expression levels were decreased significantly by XAV939 treatment, while the expression of a neurogenic transcription factor NeuroD increased in both XAV939-treated Cdo +/+ and Cdo −/− cells, compared with the control cells ( Fig. 2e ). In addition, XAV939 treatment enhanced β-tubulin III-positive cell numbers in both cell types ( Fig. 2f,g ). These data suggest that enhanced Wnt signalling caused by Cdo depletion contributes to reduced neuronal differentiation. 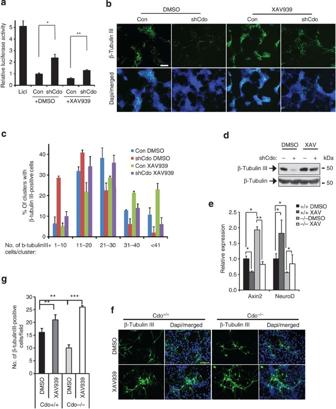Figure 2: Inhibition of Wnt signalling restored neuronal differentiation of Cdo-deficient cells. (a) Luciferase assays of P19 cells expressing either pSuper or Cdo shRNA treated either DMSO or XAV939. (b) Fluorescence microscopy of pSuper or Cdo shRNA expressing P19 cells at ITS1 immunostained with β-tubulin III antibodies. Size bar=100 μm. (c) Quantification of the representative experiment shown inb. P19 clusters that possess various numbers of β-tubulin III-positive cells were counted and plotted as percentile. More than 6 fields and at least 10 clusters/field were counted. Data are means±s.d. (n=6). (d) Immunoblot analysis of cell lysates from P19/pSuper or P19/shCdo treated with XAV939 or the vehicle DMSO in the ITS medium for 24 h. (e) qPCR with RNAs isolated from primary neurospheres ofCdo+/+orCdo−/−NPCs treated with either DMSO or 4 μM XAV939 for 24 h in the absence of bFGF. (f) Confocal microscopy ofCdo+/+andCdo−/−NPCs treated with DMSO or 4 μM of XAV939 for 24 h on the differentiation day 1, followed by immunostaining for β-tubulin III. Size bar=50 μm. (g) Quantification of the relative signal intensity of β-tubulin III from data shown inf. The mean values of at least 10 fields. Values are means±s.d. from the determinants of triplicates. All experiments in this figure were repeated three times with similar results. *P<0.05, **P<0.01, ***P<0.005. Statistical significance was tested by a Studentt-test. Figure 2: Inhibition of Wnt signalling restored neuronal differentiation of Cdo-deficient cells. ( a ) Luciferase assays of P19 cells expressing either pSuper or Cdo shRNA treated either DMSO or XAV939. ( b ) Fluorescence microscopy of pSuper or Cdo shRNA expressing P19 cells at ITS1 immunostained with β-tubulin III antibodies. Size bar=100 μm. ( c ) Quantification of the representative experiment shown in b . P19 clusters that possess various numbers of β-tubulin III-positive cells were counted and plotted as percentile. More than 6 fields and at least 10 clusters/field were counted. Data are means±s.d. ( n =6). ( d ) Immunoblot analysis of cell lysates from P19/pSuper or P19/shCdo treated with XAV939 or the vehicle DMSO in the ITS medium for 24 h. ( e ) qPCR with RNAs isolated from primary neurospheres of Cdo +/+ or Cdo −/− NPCs treated with either DMSO or 4 μM XAV939 for 24 h in the absence of bFGF. ( f ) Confocal microscopy of Cdo +/+ and Cdo −/− NPCs treated with DMSO or 4 μM of XAV939 for 24 h on the differentiation day 1, followed by immunostaining for β-tubulin III. Size bar=50 μm. ( g ) Quantification of the relative signal intensity of β-tubulin III from data shown in f . The mean values of at least 10 fields. Values are means±s.d. from the determinants of triplicates. All experiments in this figure were repeated three times with similar results. * P <0.05, ** P <0.01, *** P <0.005. Statistical significance was tested by a Student t -test. Full size image Cdo made a complex with Lrp6 and impeded Top-flash activity Since both Cdo and Lrp6 were simultaneously induced in P19 cells upon RA treatment, we examined a possible physical interaction between Cdo and Lrp6 in 293T cells by immunoprecipitation. Cdo and Lrp6 were co-immunoprecipitated when coexpressed ( Fig. 3a,b ). To assess whether Cdo and Lrp6 formed complexes endogenously, P19 cell lysates from RA1 were subjected to immunoprecipitation with either control rabbit IgG or rabbit Cdo antibodies. Lrp6 proteins were precipitated with Cdo antibodies, while no Lrp6 proteins were detected in precipitates with the control IgG ( Fig. 3c ). This interaction of Cdo with Lrp6 appeared to be specific, since two related proteins Ldlr and Lrp5 did not co-precipitate with Cdo in P19 cells ( Fig. 3d,e ). In addition, Lrp6 was co-immunoprecipitated with Cdo from brain extracts of E11.5 embryos ( Fig. 3f and Supplementary Note 2 ). Furthermore, Cdo overexpression could suppress the Top-flash activity induced by Lrp6 overexpression in 10T1/2 cells ( Fig. 3g ). These data suggest that Cdo and Lrp6 can form a complex in P19 cells and embryonic forebrain, thereby suppressing Wnt signalling. 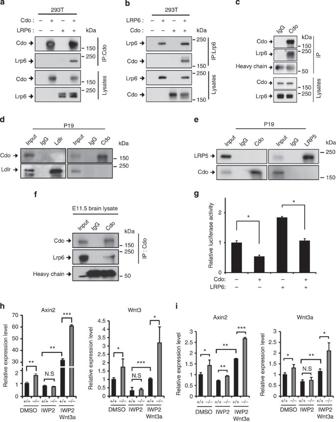Figure 3: Cdo formed a complex with Lrp6. (a,b) 293T cells were transfected with expression vectors for Cdo and Lrp6 as indicated, and lysates were subjected to immunoprecipitation with Cdo antibodies (a) or Lrp6 antibodies (b), followed by immunoblotting. (c) Lysates of P19 cells at RA1 were subjected to immunoprecipitation with control rabbit IgG or Cdo antibodies, followed by immunoblotting. (d) Co-immunoprecipitation of P19 cell lysates at G with control rabbit IgG, Cdo or Ldlr antibodies. (e) Co-immunoprecipitation of P19 cell lysates at G with control rabbit IgG, Cdo, control goat IgG or Lrp5 antibodies. (f) Extracts from embryonic brains at E11.5 were subjected to immunoprecipitation with control rabbit IgG or Cdo antibodies, followed by immunoblotting. (g) Top-flash reporter activity of 10T1/2 cells expressing Cdo or Lrp6. These values are the determinants of triplicates. Values are means±s.d. (n=3). **P<0.005. Statistical significance was tested by a Student’st-test. All experiments were repeated three times with similar results. (h) qPCR analysis ofCdo+/+orCdo−/−MEFs treated with either DMSO or 2 μM IWP2 in combination with either BSA or 20 ng per ml Wnt3a for 18 h. (i) qPCR with RNAs isolated from primary neurospheres ofCdo+/+orCdo−/−NPCs treated with either DMSO or 2 μM IWP2 in combination with either BSA or 20 ng per ml Wnt3a for 18 h after 1 day of bFGF removal. *P<0.05, **P<0.01, ***P<0.005. Statistical significance was tested by a Studentt-test. Figure 3: Cdo formed a complex with Lrp6. ( a , b ) 293T cells were transfected with expression vectors for Cdo and Lrp6 as indicated, and lysates were subjected to immunoprecipitation with Cdo antibodies ( a ) or Lrp6 antibodies ( b ), followed by immunoblotting. ( c ) Lysates of P19 cells at RA1 were subjected to immunoprecipitation with control rabbit IgG or Cdo antibodies, followed by immunoblotting. ( d ) Co-immunoprecipitation of P19 cell lysates at G with control rabbit IgG, Cdo or Ldlr antibodies. ( e ) Co-immunoprecipitation of P19 cell lysates at G with control rabbit IgG, Cdo, control goat IgG or Lrp5 antibodies. ( f ) Extracts from embryonic brains at E11.5 were subjected to immunoprecipitation with control rabbit IgG or Cdo antibodies, followed by immunoblotting. ( g ) Top-flash reporter activity of 10T1/2 cells expressing Cdo or Lrp6. These values are the determinants of triplicates. Values are means±s.d. ( n =3). ** P <0.005. Statistical significance was tested by a Student’s t -test. All experiments were repeated three times with similar results. ( h ) qPCR analysis of Cdo +/+ or Cdo −/− MEFs treated with either DMSO or 2 μM IWP2 in combination with either BSA or 20 ng per ml Wnt3a for 18 h. ( i ) qPCR with RNAs isolated from primary neurospheres of Cdo +/+ or Cdo −/− NPCs treated with either DMSO or 2 μM IWP2 in combination with either BSA or 20 ng per ml Wnt3a for 18 h after 1 day of bFGF removal. * P <0.05, ** P <0.01, *** P <0.005. Statistical significance was tested by a Student t -test. Full size image It was previously suggested that Wnt signalling activities are required for the expression of Wnt3 and Wnt3a in P19 cells during mesodermal cell differentiation, suggesting the existence of a positive feedback loop [25] , [26] . In agreement with these observations, the level of Wnt3 and Wnt3a was decreased in P19 cells treated with XAV939 (4 μM) at RA1, while Wnt3 and Wnt3a expression was enhanced by the Wnt pathway activator TWS119 (0.6 μM) treatment ( Supplementary Fig. 3a,b ). To further define the regulatory mechanism of Wnt signalling by Cdo, we utilized IWP-2, a Wnt secretion blocker, to minimize the contribution of endogenous Wnt production in Wnt signalling activation [27] in Cdo-deficient cells and analysed the response to exogenous Wnt3a treatment. To remove the residual Wnts in the culture media, Cdo +/+ and Cdo −/− MEFs were washed before the treatment with vehicle DMSO or with 2 μM IWP2 alone or in combination with either BSA or 20 ng ml −1 Wnt3a for 18 h. The IWP2 treatment reduced the expression of Axin2 and Wnt3 almost to the control level in Cdo −/− MEFs, suggesting that the endogenous Wnt signalling is needed to activate Wnt signalling. The addition of IWP2 and exogenous Wnt3a enhanced dramatically the expression of Axin2 in both cell types; however, Cdo −/− cells displayed a two-fold increase relative to the wild-type cells ( Fig. 3h ). The expression of Wnt3 was also restored in Cdo +/+ MEFs to the control level by Wnt3a treatment, while Cdo −/− MEFs displayed a stronger induction of Wnt3 expression ( Fig. 3h ). Furthermore, similar experiments were performed with Cdo +/+ and Cdo −/− NPCs. To avoid any cytotoxic effect, NPCs were treated with IWP2 for 18 h after 1 day of bFGF removal (D1). The Axin2 and Wnt3a expressions were slightly decreased when endogenous Wnt ligands were deprived by the IWP2 treatment and the addition of exogenous Wnt3a restored the expressions of Axin2 and Wnt3a to similar or higher levels to the control levels in both cell types; however, Cdo −/− NPCs showed a stronger response to Wnt3a ( Fig. 3i ). Taken together, these data suggest that Cdo deficiency can stimulate Wnt signalling both at the signal reception level and by the promotion of Wnt-signalling-dependent induction of Wnt ligands. Cdo-Lrp6 required the second Ig of Cdo and LDLR of Lrp6 To assess the interaction between Cdo and Lrp6 in detail, we attempted to identify the Cdo domain(s) mediating this interaction. Since the cytoplasmic domain of Cdo did not interact with Lrp6 ( Fig. 4a ), we then asked whether Cdo binds to Lrp6 via its ectodomain. The Cdo ectodomain consists of five Ig domains and three fibronectin III (FNIII) repeats (Fig. 4b ). We have utilized various fusion proteins of Cdo to the Fc region of human IgG gamma as described below: Cdo(Fc); the entire ectodomain fused to Fc, Ig1-5(Fc); Fc fusion protein containing Ig domains from 1 through 5, FNI-III(Fc); Fc fusion protein harbouring FNIII repeats from I through III. Since Cdo and Boc share high homologies with more than 40% sequence identities in their ectodomains, whereas Neogenin has relatively low identity with Cdo, these proteins were used as controls. The expression vectors for Fc fusion proteins as indicated were co-transfected with Lrp6 into 293T cells followed by protein A-agarose-pull down and immunoblotting. Cdo(Fc) and Ig1-5(Fc) displayed a strong interaction with Lrp6, while FNI-III(Fc) interacted only weakly with Lrp6 ( Fig. 4b ). In addition, Boc(Fc) also interacted weakly with Lrp6, while Neogenin(Fc) did not show any detectable binding to Lrp6. Surprisingly, the full-length Neogenin interacted with Lrp6 in 293T cells when overexpressed, unlike the soluble ectodomain of Neogenin ( Supplementary Fig. 4 ), suggesting that this interaction is mediated by the cytoplasmic domain of Neogenin or the Neogenin ectodoamin may achieve a distinct conformation or high density when associated with the membrane, perhaps in lipid rafts [28] . In addition, we have analysed Cdo binding to Lrp6 in the presence of Patched1 (Ptc1). To do so, 293T cells were co-transfected with Lrp6(Fc), Cdo and three varying amounts (1, 2 or 3 μg) of flag-tagged Ptc1, followed by the protein A pulldown ( Supplementary Fig. 5 ). The interaction of Cdo with Lrp6(Fc) was gradually decreased in 293T cells with increasing Ptc1 expression levels, suggesting that Lrp6 and Ptc1 undergo a steric hindrance on Cdo. 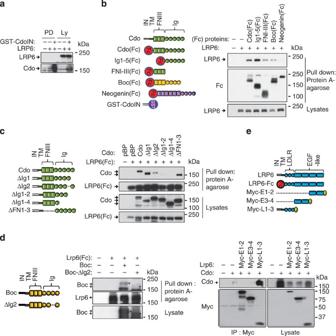Figure 4: The interaction between Cdo and Lrp6 was mediated by the second immunoglobulin of Cdo and LDLR domains of Lrp6 in the ectodomain. (a) Lysates of 293T cells co-transfected with Lrp6 and expression vectors for either a control or the fusion protein of Cdo’s intracellular region to GST (GST-CdoIN) were subjected to a pull-down assay with glutathione–agarose beads and analysed by immunoblotting. (b) Protein A-agarose pull-down assays of 293T cells co-transfected with expression vectors for Lrp6 and various Fc fusion proteins containing the ectodomain of Cdo, Boc or Neogenin. (c) Protein A-agarose pull-down assays of 293T cells transfected with expression vectors for a Lrp6 ectodomain–Fc fusion protein Lrp6 (Fc) and various Cdo deletion mutants. (d) Protein A–agarose pull-down assays of 293T cells co-transfected with Lrp6 (Fc) and the full length or Ig2 deletion mutant of Boc. (e) Co-immunoprecipitation of 293T cell lysates transfected with expression vectors for Cdo and three different myc-tagged Lrp6 extracellular domains; EGF-like domains 1–2 (E1–2), E3–4 or LDLR domain (L1–3) with a myc antibody. All experiments were repeated at least three times with similar results. Figure 4: The interaction between Cdo and Lrp6 was mediated by the second immunoglobulin of Cdo and LDLR domains of Lrp6 in the ectodomain. ( a ) Lysates of 293T cells co-transfected with Lrp6 and expression vectors for either a control or the fusion protein of Cdo’s intracellular region to GST (GST-CdoIN) were subjected to a pull-down assay with glutathione–agarose beads and analysed by immunoblotting. ( b ) Protein A-agarose pull-down assays of 293T cells co-transfected with expression vectors for Lrp6 and various Fc fusion proteins containing the ectodomain of Cdo, Boc or Neogenin. ( c ) Protein A-agarose pull-down assays of 293T cells transfected with expression vectors for a Lrp6 ectodomain–Fc fusion protein Lrp6 (Fc) and various Cdo deletion mutants. ( d ) Protein A–agarose pull-down assays of 293T cells co-transfected with Lrp6 (Fc) and the full length or Ig2 deletion mutant of Boc. ( e ) Co-immunoprecipitation of 293T cell lysates transfected with expression vectors for Cdo and three different myc-tagged Lrp6 extracellular domains; EGF-like domains 1–2 (E1–2), E3–4 or LDLR domain (L1–3) with a myc antibody. All experiments were repeated at least three times with similar results. Full size image To determine the responsible Ig domain(s) of Cdo for Lrp6 binding, various deletion mutants of Cdo’s ectodomain were co-transfected with Lrp6(Fc), a fusion protein of Lrp6’s ectodomain to Fc, and lysates were subjected to protein A-agarose pulldown. The deletion mutants for the first Ig domain (ΔIg1) and the entire fibronectin domain (ΔFNI-III) displayed the equivalent interaction capability to the full-length Cdo, while Cdo deletion mutants harbouring the deletion of the second Ig domain (ΔIg2, ΔIg1–2, ΔIg1–4) exhibited a stark reduction in Lrp6 binding ( Fig. 4c ). Since the Ig2 domain of Cdo and Boc is highly conserved, we have tested whether Boc also interacts with Lrp6 via its Ig2. As shown in Fig. 4d , Boc-ΔIg2 mutant showed a diminished interaction with Lrp6(Fc). These data suggest that the Ig2 domain of Cdo and Boc mediates the interaction with Lrp6. To further characterize, we examined the domain of Lrp6 mediating Cdo binding. The ectodomain of Lrp6 consists of four EGF and three LDLR repeats ( Fig. 4e ). Since the flag-tagged EGF1-4 deletion mutant of Lrp6 interacted with Cdo ( Supplementary Fig. 6 ), we assessed whether LDLR domains are responsible for Cdo interaction by co-transfecting three different Myc-tagged Lrp6 ectodomains, EGF1-2 (E1-2), E3-4 or LDLR1-3 (L1-3) with Cdo, followed by immunoprecipitation ( Fig. 4e ). Cdo was co-precipitated efficiently with Myc-tagged L1-3 of Lrp6, but not with EGF repeats. These data suggest that Cdo forms complexes with Lrp6 and this interaction is mediated by the second Ig domain of Cdo and the LDLR domains of Lrp6 in the ectodomain. Wnt signalling was restored with Lrp6-binding-defective Cdo To examine the function of this interaction, the effect of the expression of control pBP, full-length Cdo or the Lrp6-binding-deficient ΔIg2 on the β-catenin transactivation activity was analysed. ΔIg2 failed to suppress fully the Top-flash activity in 10T1/2 MEFs, compared with the full-length Cdo ( Fig. 5a ). To further assess its functional role in Wnt signalling and neuronal differentiation, control, Cdo or ΔIg2-expressing P19 cells were subjected to immunoblotting. Cdo overexpression reduced the level of pLrp6 and β-catenin* ~40–50% of the control, while the expression of ΔIg2 mutant failed to do so ( Fig. 5b ). To assess neuronal differentiation, P19 cells transfected with control, Cdo or ΔIg2 at ITS1 were analysed for β-tubulin III expression. P19/Cdo cells displayed an ~2.5-fold increase in β-tubulin III proteins compared with the control cells, while P19/ΔIg2 cells showed substantially lower levels of β-tubulin III than in the control cells ( Fig. 5c ). Furthermore, Cdo overexpression led to an increase in β-tubulin III-positive cells per cluster, while ΔIg2 expression failed to enhance neuronal differentiation relative to the controls ( Fig. 5d,e ). Consistent with the interaction between Boc and Lrp6, overexpression or knockdown of Boc in P19 cells decreased or increased the level of pLrp6, respectively, suggesting that Boc can suppress Wnt signalling similarly to Cdo ( Supplementary Fig. 7a ). Similarly to Cdo, Boc-ΔIg2 expression also showed an incomplete suppression of the Top-flash activity, compared with the full-length Boc ( Supplementary Fig. 7b ). These data suggest that the interaction of Cdo with Lrp6 is critical for its suppressive activity for Wnt signalling and promotion of neuronal differentiation. 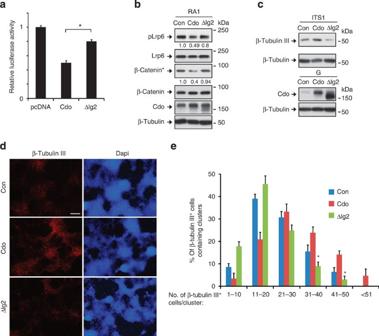Figure 5: The binding deficient Cdo mutant failed to suppress Wnt signalling. (a) Luciferase assays of 10T1/2 cells expressing control, Cdo or ΔIg2 vectors. These values are the determinants of triplicates and this experiment was repeated three times with similar results. Values are means±s.d. (n=3). *P<0.05. Statistical significance was tested by a Student’st-test. (b) pBp, Cdo or ΔIg2-transfected P19 cells were analysed by immunoblotting. Quantification of the normalized signal intensity for β-catenin* and pLrp6 relative to the total β-catenin or Lrp6 protein is shown below each lane and the signals in the control lane are set to 1. (c) pBP, Cdo or ΔIg2-transfected P19 cells were analysed by immunoblotting for Cdo expression at G and β-tubulin III at ITS1. The quantification of the normalized signal intensity for β-tubulin III relative to the loading control β-tubulin is shown below each lane and the signals in the control lane are set to 1. (d) pBp, Cdo or ΔIg2-transfected P19 cells at ITS1 were immunostained with β-tubulin III antibodies followed by fluorescence microscopy. Size bar=100 μm. (e) Quantification of the representative experiment shown ind. P19 clusters that possess various numbers of β-tubulin III-positive cells were counted and plotted as percentile. More than 10 fields and at least 10 clusters per field were counted. Data are means±s.d. (n=10). *P<0.05. Statistical significance was tested by a Student’st-test. The experiment was repeated three times with similar results. Figure 5: The binding deficient Cdo mutant failed to suppress Wnt signalling. ( a ) Luciferase assays of 10T1/2 cells expressing control, Cdo or ΔIg2 vectors. These values are the determinants of triplicates and this experiment was repeated three times with similar results. Values are means±s.d. ( n =3). * P <0.05. Statistical significance was tested by a Student’s t -test. ( b ) pBp, Cdo or ΔIg2-transfected P19 cells were analysed by immunoblotting. Quantification of the normalized signal intensity for β-catenin* and pLrp6 relative to the total β-catenin or Lrp6 protein is shown below each lane and the signals in the control lane are set to 1. ( c ) pBP, Cdo or ΔIg2-transfected P19 cells were analysed by immunoblotting for Cdo expression at G and β-tubulin III at ITS1. The quantification of the normalized signal intensity for β-tubulin III relative to the loading control β-tubulin is shown below each lane and the signals in the control lane are set to 1. ( d ) pBp, Cdo or ΔIg2-transfected P19 cells at ITS1 were immunostained with β-tubulin III antibodies followed by fluorescence microscopy. Size bar=100 μm. ( e ) Quantification of the representative experiment shown in d . P19 clusters that possess various numbers of β-tubulin III-positive cells were counted and plotted as percentile. More than 10 fields and at least 10 clusters per field were counted. Data are means±s.d. ( n =10). * P <0.05. Statistical significance was tested by a Student’s t -test. The experiment was repeated three times with similar results. Full size image Cdo knockout raised cell growth and dorsal marker expression Next, we analysed the effect of Cdo deficiency on Wnt signalling by utilizing Cdo +/− and Cdo −/− embryos carrying a Top-galactosidase Wnt-reporter (Top-Gal). Among two different alleles of Cdo mutant mice designated as Cdo LacZ1 and Cdo LacZ2 , Cdo LacZ1 mice were used since this allele shows only very weak staining for β-galactosidase [29] . Consistently, the Cdo −/− embryo on E11.5 without the Top-Gal transgene showed a very faint staining for β-galactosidase in the developing eye and the proximal region of limb buds ( Fig. 6a ). The Top-Gal activity was detected in the dorsal region of fore- and midbrain, mid-hindbrain boundary, eye, otic vesicle, craniofacial structures, the distal area of the limb bud in both Cdo +/− and Cdo −/− embryos ( Fig. 6b,d ). The intensity of Top-Gal staining was stronger in the mutant tissues where Cdo is normally expressed, especially obvious in the dorsal forebrain (enlarged in Fig. 6c,e ), midbrain and the maxillary process. In addition, it appeared to be an early developmental stage-specific event, since this effect of enhanced Top-Gal activities in the Cdo −/− forebrain was observed clearly only at early embryonic days. At later time points such as E13.5, the enhancement of Top-Gal staining was less prominent ( Supplementary Fig. 8 ). To verify the effect of Cdo deficiency on Wnt signalling in the forebrain, RNAs isolated from Cdo +/+ and Cdo −/− forebrains on E11.5 were subjected to qPCR analysis. As shown in Fig. 6f , the expression of Wnt3a, Axin2 and Gli3 in Cdo −/− forebrains was increased ~2–2.5 fold. In contrast, the expression of Shh and Ptc1 decreased to 85% and 60% of the control, respectively, while Gli1 expression levels did not change. These data further support that Wnt signalling is enhanced in the Cdo-deficient forebrain, while Shh signalling is decreased. 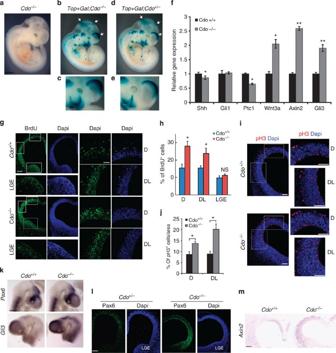Figure 6: Cdo deficiency caused an increase in cell proliferation and the expressions of dorsal telencephalic markers. (a) β-galactosidase staining of the littermate embryos with genotypes,Cdo−/−,Top-Gal;Cdo−/−andTop-Gal;Cdo+/−at E11.5. The expression domain of Top-Gal in the midbrain and forebrain are marked with arrows (b,d). The forebrain area ofCdo−/−andCdo+/−is shown in an enlarged view in the lower panels (c,e). The Top-Gal activity in the maxillary of theTop-Gal;Cdo−/−embryo is also enhanced (marked with asterisks). Size bar=1 mm. (f) qPCR analysis with RNAs isolated fromCdo+/+andCdo−/−E11.5 forebrains. Values are the determinants of triplicates. This experiment was repeated with two independent samples. (g) Coronal sections ofCdo+/+andCdo−/−forebrain at E11.5 were subjected to immunostaining for BrdU incorporation. Boxed areas labelled D (the dorsal region), DL (the dorsolateral region) and lateral ganglionic eminence (LGE) ofCdo+/+andCdo−/−forebrains. Size bar=100 μm (left), 30 μm (right). (h) Quantification of BrdU incorporation inCdo+/+andCdo−/−forebrains. BrdU-positive cells were plotted as percentile, relative to the total cell number. (i) Coronal sections ofCdo+/+andCdo−/−forebrain at E11.5 were subjected to immunostaining for pH3. The boxed areas ofCdo+/+andCdo−/−forebrains in the fluorescence images (the left panel) are shown enlarged in the right panels labelled D or DL. Size bar=100 μm. The white asterisks are marking autofluorescent red blood cells. (j) Quantification of pH3 inCdo+/+andCdo−/−forebrains. pH3-positive cells were plotted as percentile, relative to the total cell number. (k)Cdo+/+andCdo−/−embryos at E9.5 were analysed by wholemountin situhybridization for Pax6 and Gli3 expression. Size bar=500 μm. (l) Coronal sections ofCdo+/−andCdo−/−forebrain at E11.5 were subjected to immunostaining for Pax6 expression. Size bar=100 μm. (m) RNAin situhybridization for Axin2 expression with coronal sections ofCdo+/+andCdo−/−forebrain. Size bar=100 μm. *P<0.05, **P<0.01. Statistical significance was tested by a Student’st-test. All data are presented in this figure as mean±s.d. Figure 6: Cdo deficiency caused an increase in cell proliferation and the expressions of dorsal telencephalic markers. ( a ) β-galactosidase staining of the littermate embryos with genotypes, Cdo −/− , Top-Gal;Cdo −/− and Top-Gal;Cdo +/− at E11.5. The expression domain of Top-Gal in the midbrain and forebrain are marked with arrows ( b , d ). The forebrain area of Cdo −/− and Cdo +/− is shown in an enlarged view in the lower panels ( c , e ). The Top-Gal activity in the maxillary of the Top-Gal;Cdo −/− embryo is also enhanced (marked with asterisks). Size bar=1 mm. ( f ) qPCR analysis with RNAs isolated from Cdo +/+ and Cdo −/− E11.5 forebrains. Values are the determinants of triplicates. This experiment was repeated with two independent samples. ( g ) Coronal sections of Cdo +/+ and Cdo −/− forebrain at E11.5 were subjected to immunostaining for BrdU incorporation. Boxed areas labelled D (the dorsal region), DL (the dorsolateral region) and lateral ganglionic eminence (LGE) of Cdo +/+ and Cdo −/− forebrains. Size bar=100 μm (left), 30 μm (right). ( h ) Quantification of BrdU incorporation in Cdo +/+ and Cdo −/− forebrains. BrdU-positive cells were plotted as percentile, relative to the total cell number. ( i ) Coronal sections of Cdo +/+ and Cdo −/− forebrain at E11.5 were subjected to immunostaining for pH3. The boxed areas of Cdo +/+ and Cdo −/− forebrains in the fluorescence images (the left panel) are shown enlarged in the right panels labelled D or DL. Size bar=100 μm. The white asterisks are marking autofluorescent red blood cells. ( j ) Quantification of pH3 in Cdo +/+ and Cdo −/− forebrains. pH3-positive cells were plotted as percentile, relative to the total cell number. ( k ) Cdo +/+ and Cdo −/− embryos at E9.5 were analysed by wholemount in situ hybridization for Pax6 and Gli3 expression. Size bar=500 μm. ( l ) Coronal sections of Cdo +/− and Cdo −/− forebrain at E11.5 were subjected to immunostaining for Pax6 expression. Size bar=100 μm. ( m ) RNA in situ hybridization for Axin2 expression with coronal sections of Cdo +/+ and Cdo −/− forebrain. Size bar=100 μm. * P <0.05, ** P <0.01. Statistical significance was tested by a Student’s t -test. All data are presented in this figure as mean±s.d. Full size image We then examined the effect of enhanced Wnt signalling in the dorsal forebrain on cell proliferation by bromodeoxyuridine (BrdU) incorporation and phospho-histone H3 (pH3) immunostaining. BrdU-positive cells were observed throughout the neuroepithelium of Cdo +/+ and Cdo −/− embryonic telencephalons at E11.5; however, the dorsal (D) and dorsolateral areas of the Cdo −/− telencephalon contained more BrdU-positive cells than the control ( Fig. 6g,h ). This increase appeared to be specific for the dorsal forebrain, since the lateral ganglionic eminence (LGE) that does not express Cdo exhibited no difference ( Fig. 6g,h ). Consistently, the D and dorsolateral areas of Cdo −/− telencephalon contained more pH3-positive cells, compared with the wild type ( Fig. 6i,j ). In addition, we did not observe any signs of overt cell death analysed by the cleaved Caspase3 immunostaining ( Supplementary Fig. 9 ). To determine whether enhanced Wnt signalling in the Cdo −/− telencephalon alters the dorsoventral patterning, we analysed expressions of two dorsal regulators, Gli3 and Pax6, in Cdo +/+ and Cdo −/− embryos on E9.5 by whole mount in situ hybridization ( Fig. 6k ), the expression of Pax6 protein in Cdo +/− and Cdo −/− at E11.5 by immunostaining ( Fig. 6l ) and the expression of Axin2 expression by in situ hybridization ( Fig. 6m ). Pax6 and Gli3 were expressed robustly in the dorsal area of the telencephalon as seen in Cdo +/+ embryos, while Pax6 and Gli3 expression was enhanced dorsally as well as expanded ventrally in Cdo −/− embryos. Similarly, the expression of Pax6 protein and Axin2 mRNA was also enhanced dorsally and expanded ventrally into the portion of the LGE in Cdo −/− telencephalon, compared with control embryos. These data suggest that Cdo deficiency enhances Wnt signalling in addition to reducing Shh signalling and thereby contributes to dorsalization of the developing telencephalon. Taken together, our data suggest that Cdo suppresses Wnt signalling via multiple mechanisms, including direct Lrp6 binding via its Ig2 domain, and production of Wnts. In the absence of Cdo, Wnt signalling is enhanced at the signal reception, likely through increased Lrp6–Fz interaction, which may in turn increase Wnt expression levels as part of feedback regulation, thereby regulating neuronal differentiation and early forebrain development. In this study, we provide lines of evidence for a functional interaction between Cdo and Lrp6, a co-receptor for Wnt signalling, that results in Wnt signalling suppression and promotion of neuronal differentiation. On the basis of our previous and current work, we propose that Cdo promotes cell differentiation in multiple ways, including inhibition of Wnt signalling and activation of the key neurogenic transcription factors through Bnip2/p38MAPK signalling [30] , [31] . Although cadherin ligation initiates Cdo-mediated p38MAPK signalling to promote differentiation of skeletal myoblasts, the initiating signals for Cdo/p38MAPK in neural precursors are as yet unknown. Cdo appears to work as a multifunctional component of several receptor complexes mediating signals from cell adhesion molecules, netrins and Shh [30] , [31] , [32] . All previously characterized receptor interactions are mediated by the FNIII repeats in the Cdo ectodomain. N-cadherin binds the first FNIII domain (FN1), whereas Gas1, another Shh co-receptor, interacts with FN2 (refs 15 , 30 ). The primary Shh receptor Patched1 interacts with FN1-2, whereas Shh itself binds the FN3 repeat [23] , [33] . Finally, the netrin receptor Neogenin also binds to FN3 (R. Krauss, personal communication). Our findings identify, for the first time, a functional role for the Cdo Ig repeats, specifically Ig2. It is of interest that Ig2 is, after the FNIII repeats, the most evolutionarily conserved repeat among this subfamily, which includes the vertebrate othologue Boc and the Drosophila proteins Ihog and Boi [34] . Consistently, Boc also interacts with Lrp6 via Ig2. Therefore, Ihog/Boi may interact with Arrow, the fly orthologue of Lrp5/6, to regulate Wnt signalling in specific contexts. Although Lrp5 and Lrp6 share a high sequence homology in their extracellular domains, we failed to detect Lrp5 interaction with Cdo. Since the interaction of Lrp6 with Cdo is mediated by its LDLR domains, which exhibit lower sequence homology than the EGF repeats and contain more glycosylation sites than Lrp5 (ref. 35 ), this may contribute to the binding specificity of Lrp6 with Cdo. It will be of interest to investigate in future the significance of this regulatory mechanism in the divergent function of Lrp5/6 in vivo . Since the LDLR domains mediate Lrp6 dimerization required for robust Wnt signalling [36] , it will be interesting to investigate whether Cdo interferes with Lrp6 dimerization to prevent Wnt signalling activation. Cell–cell contact-initiated signalling through N-cadherin complexes has been implicated in inhibition or activation of Wnt signalling by sequestration of β-catenin or by Akt-dependent phosphorylation of β-catenin, leading to inhibition or activation of its transcriptional activity, respectively. In the developing cortical plate, N-cadherin can form a complex with Lrp6 to activate Wnt signalling, thereby promoting proliferation of NPCs [37] , [38] . Moreover, inhibition of cell–cell contact-based signalling results in premature neuronal differentiation [38] . It is plausible that Cdo forms ternary complexes with Lrp6 via its Ig2 repeat and with N-cadherin via its FN1 to inhibit Wnt signalling. Further studies will be required to address whether such higher-order complexes are required for Cdo-mediated inhibition of Wnt signalling, or whether a simple model, whereby Cdo sequesters Lrp6 from other Wnt signalling components may be operative. Cdo is required for the full Shh signalling activity to ventralize the forebrain and to counteract dorsalization signals such as Wnt. The ventral expansion of Gli3, Pax6 and Axin2 in Cdo-deficient forebrains may be largely because of the weakened Shh signalling from the ventral forebrain. However, several observations indicate that Cdo more directly regulates Wnt signalling. First, Cdo is highly expressed in the dorsal region of the early developing CNS, where Shh signalling is absent [39] . Second, the enhanced expression levels of Axin2, Gli3 and Pax6 in the dorsal forebrain of Cdo mutant embryos are likely because of enhanced Wnt signalling, since Shh is not expressed in the dorsal forebrain at this time point. Third, Shh signalling is not grossly affected in Cdo-depleted P19 cells in the early stages of neurogenesis, a time point when Wnt signalling is upregulated as well as the modulation of Shh signalling by the treatment with an activator or inhibitor does not specifically affect Wnt signalling ( Supplementary Fig. 10a–c ). Last, the ΔIg2 Cdo mutant is still competent for Shh signalling [23] . Interestingly, it has recently been reported that Ihog/Boi interact with Shifted, a fly orthologue of the Wnt signalling inhibitor Wif1, to stimulate hedgehog signalling via interaction with the hedgehog receptor complex [40] . In addition, Ihog enhances the Wnt inhibitory activity of Wif1. Although whether such an interaction occurs in vertebrate systems is uncharacterized, it is conceivable that Cdo may also suppress Wnt signalling via interaction with Wif1. However, it appears to be less likely that Wif1 interaction is a major mechanism by which Cdo suppresses Wnt signalling, since Wif1 overexpression in P19 cells affected only weakly Wnt signalling ( Supplementary Fig. 10d,e ). On the basis of the ubiquitous expression pattern of Lrp6 in developing embryo [41] and Ptc1’s interference with Cdo binding to Lrp6, it is tempting to speculate that individual Cdo complexes may only be able to regulate Wnt or Hh signalling, depending on whether they contain Lrp6 or Ptc1. While Cdo can dampen Wnt signalling dorsally by binding Lrp6, Lrp6 may be able to indirectly regulate Shh signalling ventrally by controlling the access of Cdo to Ptc1. Further studies will be required to address whether such counteracting mechanism exists. These findings support the notion that Cdo functions as a co-receptor shared by multiple pathways [42] to regulate spatiotemporal signalling between N-cadherin, Wnt and Shh signalling in embryonic development. Cell cultures and immunocytochemistry P19, 10T1/2 and 293T cells were purchased from ATCC, and C17.2 neuronal progenitor cells were purchased form Sigma-Aldrich. These cells were cultured as previously described [20] . P19 cells were cultured in α-minimum essential medium supplemented with 10% fetal bovine serum (Invitrogen) and 1% penicillin and streptomycin, which was referred as G in this study. To induce neuronal differentiation of these cells, 3 × 10 5 cells per 60 mm poly- L -lysine (PLL)-coated plastic dish were seeded and, 24 h later, treated with 0.5 μM all-trans-RA (Sigma) in DMEM/F12 medium supplemented with insulin-transferrin-selenium (Invitrogen; referred as ITS throughout the manuscript) for 2 days followed by switching into DMEM/F12/ITS in the absence of RA with fresh medium replacement every 2 days. To modulate Wnt signalling activities, we have treated P19 cells with an inhibitor XAV939 (4 μM, Selleck Chem) and an activator TWS119 (0.6 μM, Calbiochem) at RA1. To inhibit endogenous Wnt ligand secretion, we have treated MEFs and NPCs with an IWP2 (2 μM, Calbiochem) for 18 h before cell harvest. To modulate Shh signalling, P19 cells were treated with either an inhibitor Sant1 (50 μM, Santa Cruz Biotechnology) or an activator Purmorphamine (2 μM, Calbiochem). Isolation and maintenance of MEFs from Cdo +/− and Cdo −/− mice were followed essentially by standard protocols [30] . Briefly, the bodies of E13.5 embryos harvested from intercrosses of heterozygous mice were minced and trypsinized for 2–3 min followed by trituration. MEFs were then centrifuged and resuspended in DMEM medium with 10% fetal bovine serum. MEFs were immortalized by successive passaging of 3–6 × 10 5 cells every 2 days. In this study, we have used MEFs from the passage number 35–40. Isolation and culture of NPCs were performed similarly as previously described [13] . In this study, forebrains of E12 embryos from the time-mating of the Cdo +/ − mice were utilized. To induce differentiation of NPCs, neurospheres were cultured for 2–3 days without bFGF (designated D2 and D3) in DMEM/F12 medium containing N2/B27 supplements (Invitrogen), followed by immunoblotting and qPCR analyses. To examine the effect of Wnt3a on NPCs, neurospheres were dissociated as single cells with Versene and plated on poly- L -lysine-coated chamber slides, followed by 20 ng ml −1 Wnt3a (R&D systems) treatment for 24 h at D2. Then cells were fixed and immunostained with β-catenin antibodies, followed by observation with confocal microscopy. Immunostaining of P19, 10T1/2 cells and NPCs was carried out as previously described [19] . Briefly, for β-tubulin III staining, P19 cells were induced to differentiate for 3 days, fixed and immunostained with anti-β-tubulin III antibodies (1:250). For β-catenin staining, NPCs were induced to differentiate for 2 days with BSA or Wnt3a. Cells were fixed, permeabilized with 0.5% triton X-100 (Sigma) for 15 min at room temperature and immunoreacted with mouse anti-β-catenin antibody overnight (1:250). Then, incubation with secondary florescence antibodies was performed for 1 h at RT. The used secondary florescence antibodies are listed below; Alexa Fluor 488 goat anti-mouse antibody, Alexa Fluor 594 goat anti-mouse antibody and Alexa Fluor 594 goat anti-rabbit antibody (1: 500, Invitrogen). Fluorescence microscopy was performed with the help of Nikon ECLIPS TE-2000U and NIS-Elements F software (Nikon). Confocal microscopy was performed at SKKU School of Medicine-Microscopy Shared Resource Facility with Zeiss LSM-510, LSM-710 Meta confocal microscope. Protein analysis and antibodies Western blot analyses were carried out as described previously [32] . Briefly, transferred membranes were blocked with 5% skim milk in TBST (10 mM Tris–HCl, pH 8.0, 150 mM NaCl, 0.1% Tween-20) for 30 min and incubated with primary antibodies at 4 °C for overnight. Primary antibodies used in this study were as follows: Cdo (1:1,000) from R&D Systems; β-tubulin III (1:2,000) from Sigma; β-catenin (1:1,000) from BD Transduction Laboratories; Active β-catenin (1:500) from Millipore; CREB (1:1,000), GSK-3β (1:1,000), pGSK-3β (1:1,000) and p-Histone H3 (pH3, 1: 500) from Cell Signaling; Pax6 (1:500), α-tubulin (1:1,000), Lamin B1(1:1,000), Lrp6(1:1,000) and pLrp6 (1:500) from Abcam; Lrp5(1:2,000), Cyclin D1 (1:1,000) and Ldlr (1:2,000) from Santa Cruz; β-tubulin (1:2,000) and N-cadherin (1:1,000) from Invitrogen; α-Flag (1:1,000), α-Myc (1:500) and α-HA (1:1,000) from Abfrontier; BrdU (1:1,000) from Chemicon. For co-immunoprecipitation (co-IP), each plasmid construct was transcfected into the 293T cell using Lipofectamine 2000 (Invitrogen). To examine Lrp6-Cdo complex formation, co-IP assays were performed as previously described [16] . The constructs for Cdo-deletion mutants lacking various ectodomain repeats, Cdo-GST, Cdo-Fc, Boc-Fc and Neogenin-Fc, were previously described [16] . The constructs for Lrp6 deletion mutants were previously described [43] . The human Wif1(HA) construct was kindly provided by Dr CS Shin (Seoul National University). The human Lrp6(Fc) construct was purchased from Addgene. For the co-IP of Boc with Lrp6, the full-length Boc and ΔIg2-Boc plasmids were kindly provided by Dr B. Allen (University of Michigan). For the nuclear fractionation assay, P19 cells or MEF pellets were resuspended in 100 μl of Buffer A (40 mM Tris–HCl at pH 7.4, 10 mM NaCl, 1 mM EDTA, 1 mM dithiothreitol (DTT) and protease inhibitors) and incubated on ice for 15 min. After the addition of 7.5 μl 10% NP-40, cells were briefly vortexed and centrifuged at 133,000 r.p.m. at 4 °C for 10 min. After transferring the cytoplasmic supernatant, the remaining pellets were resuspended in 50 μl Buffer B (40 mM Tris–HCl at pH 7.4, 420 mM NaCl, 10% glycerol, 1 mM EDTA, 1 mM DTT and proteinase inhibitors) followed by incubation for 20 min on ice and a subsequent cold centrifugation with 133,000 r.p.m. for 10 min. The supernatant containing the nuclear fraction was transferred into a new tube, and the fractions were analysed by immunoblotting. For controls, we have utilized α-tubulin as a cytosolic marker and Lamin B1 and CREB as nuclear markers. RNA analysis Total RNAs from cells and tissues were prepared using easy-BLUE reagent (Intron biotechnology). cDNA was generated with 0.5 μg of total RNA as templates by using the PrimeScript RT reagent kit (TaKaRa) according to the manufacturer’s instructions. qRT–PCR was performed as described previously [44] . Briefly, qPCR reactions were carried out using SYBR premix Ex Taq (TaKaRa) and Thermal Cycler Dice Real Time System (TP800, TaKaRa) according to the manufacturer’s instructions. Gapdh was used as an internal control. Primer sequences used in this study were as follows: Wnt1 F; 5′- CTCAGACACACTCGCTGGTC -3′, R; 5′- TACATCAGGAACCGCAACAC -3′ Wnt3 F; 5′- GCCGACTTCGGGGTGCTGGT -3′, R; 5′- CTTGAAGAGCGCGTACTTAG -3′ Wnt3a F; 5′- TAACACGGGAGCAGGGTTCAT -3′, R; 5′- AAGGGGGTCTCCAAAAGTTCC -3′ Wnt5a F; 5′- TCCTATGAGAGCGCACGCAT -3′, R; 5′- CAGCTTGCCCCGGCTGTTGA -3′ β-tubulin III F; 5′- CAACGTCAAGGTAGCCGTGT -3′, R; 5′- TCCGATTCCTCGTCATCATC -3′ Cdo F; 5′- GTGTGCTTGGGGTTATGGTC -3′, R; 5′- CTCCATTTATGTTTCCACTC -3′ Gapdh F; 5′- ACCACAGTCCATGCCATCAC -3′, R; 5′- TCCACCACCCTGTTGCTGTA -3′ Axin2 F; 5′- AGTGAGACGCTCTCCCTCACCA -3′, R; 5′- GAAACGCGCATAGGTTTGCTGGAC -3′, Wif1 F; 5′- GAGGAAAGCCCAACAAAAA -3′, R; 5′- ACACAGACCACCGTTCATAC -3′, Shh F; 5′- CTGGCCAGATGTTTTCTGGT -3′, R; 5′- GATGTCGGGGTTGTAATTGG -3′, Gli1 F; 5′- CCAAGCCAACTTTATGTCAGGGR -3′; 5′- AGCCCGCTTCTTTGTTAATTTGA , Dkk1 F; 5′- TCGGAGATGATGGTTGTGTG -3′, R; 5′- GCAAGGGTAGGGCTGGTAGT -3′, Gli3 F; 5′- AGCAACCAGGAGCCTGAAGTC -3′, R; 5′- GTCTTGAGTAGGCTTTTGTGC -3′, Neuro D F; 5′- TGACCTTTCCCATGCTGAAT -3′, R; 5′- AAGTGCTAAGGCAACGCAAT -3′ Patched1 F; 5′- TTTTGGTTGTGGGTCTCCTC -3′, R; 5′- TCCACCGTAAAGGAGGCTTA -3′ Reporter assay P19, 10T1/2 and MEF cells were transiently co-transfected with 8 × Top-flash reporter construct (Addgene) and RSV-β-galactosidase as an internal control plus either control shRNA, Cdo, shCdo or Boc expression vectors using Lipofectamine 2000. Twenty-four hours later, cells were switched either into serum-free medium supplemented with 0.5 μM all- trans -RA (Sigma-Aldrich) for P19 cells or 2% horse serum containing medium for 10T1/2 and MEFs. After the additional 24 h, cells were harvested and the luciferase activity was analysed according to the manufacturer’s instruction (Promega) and normalized by the β-galactosidase internal control. Mice, β-Gal staining and BrdU assay Cdo +/− mice were maintained on a C57BL/6 background and Top-Gal transgenic mice were purchased from The Jackson Laboratory and maintained on CD1 background. All animal studies were reviewed and approved by the International Animal Care and Use Committee of SKKU School of Medicine (SUSM). SUSM is an Association for Assessment and Accreditation of Laboratory Animal Care international accredited facility and abides by the Institute for Laboratory Animal Research guide. For wholemount β-Gal staining of Top-Gal;Cdo +/− and Top-Gal;Cdo −/− embryos, Cdo +/− mice were mated with Top-Gal mice and embryos at E11.5 were harvested followed β-galactosidase staining essentially as previously described [13] with the exception that fixation time was for 1 h at 4 °C. Images were taken with Nikon SMZ-1500 microscope. To monitor cell proliferation, BrdU incorporation was performed as previously described [13] . Briefly, time-mated pregnant mice were injected with 100 mg BrdU (Sigma) per gram of body weight and, 2 h later, dissected embryos were fixed in 4% paraformaldehyde followed by embedding in paraffin and sectioning at 7 μm. For immunohistochemistry, sections were immunostained either with antibodies to BrdU, pH3 or Pax6. For nucleus staining, samples were incubated in 4 μM of 4′,6-diamidino-2-phenylindole in PBS for 5 min (BD Biosciences). Zeiss LSM-510 Meta confocal and Axiophot2 fluorescence microscopes were used for imaging. RNA in situ hybridization RNA in situ hybridization of E9.5 and E11.5 mouse embryo was carried out as previously described [13] , [20] . Briefly, for wholemount in situ hybridization, fixed and dehydrated E9.5 embryos were rehydrated into PTW buffer (0.1% Tween-20 in PBS) and bleached with 6% hydrogen peroxide (H 2 O 2 ) in PTW. After several times of washing, embryos were treated with 10 μg per ml proteinase K in PTW for 20 min. Embryos were then rinsed, postfixed and equilibrated in the hybridization solution (50% formamide, 1.3 × SSC, 5 mM EDTA, 50 μg per ml yeast tRNA, 0.2% Tween-20, 0.5% Chaps, 100 μg per ml heparin) at 65 °C. Embryos were incubated with digoxygenin-labelled probe in hybridization solution overnight at 65 °C. After the extensive washing, the embryos were blocked and incubated overnight at 4 °C with alkaline-phosphatase-conjugated anti-digoxygenin antibody (Roche) in blocking buffer containing 2% Blocking Reagent (Roche), 20% heat-inactivated sheep serum in Washing solution I (100 mM maleic acid at pH 7.5, 150 mM NaCl, 0.1% Tween-20). After washing the embryos with Washing solution I and Washing solution II (500 mM NaCl, 100 mM Tris/HCl (pH 9.5), 50 mM MgCl 2 , 1% Tween-20), signals were developed using the BM Purple AP substrate (Roche). For RNA in situ hybridization, deparaffinized E11.5 embyro sections were rehydrated and incubated in 6% H 2 O 2 in PBS for 15 min to bleaching endogenous peroxidase activity. After three times of PBS washing, the sections were treated with 10 μg per ml protease K in PBS for 10 min. To inhibit residual protease K activity, 0.2% of fresh glycine in PBS were treated. Sections were refixed and acetylated with 0.25% of acetic anhydride (Sigma) in 100 mM Tris (pH 7.5). After washing with 2 × SSC buffer, the sections were dehydrated by serial incubation of ethanol solutions (30–100%) followed by air-drying. Sections were then incubated with hybridization mix (4 μg of digoxygenin-labelled Axin 2 probe (kindly provided by Dr F. Constantini), 3.3 × SSC (pH 5.0), 33% formamide, 3.3% blocking (Roche), 6.6% Dextran sulfate, 3.3 mM EDTA, 0.06% Tween-20, 60 μg Heparin and 100 μg Yeast tRNA) overnight at 65 °C with 5 ml of soaking solution (1 ml of 20 × SSC pH 7.5, 2.5 ml of formamide and 1.5 ml of ddH 2 O). After serial washes with SSC and TES buffer (0.5 M NaCl, 10 mM Tris HCl (pH 8.0), 5 mM EDTA), the sections were blocked and incubated at 4 °C for 2 h following anti-DIG-AP antibody incubation overnight at 4 °C. Signals were developed in the same way as in wholemount in situ hybridization. Statistical analysis Statistical analyses of the results are expressed as mean±s.d. from at least three independent experiments. Error bars represent means±s.d. For comparison between multiple groups, statistical significance was tested by a Student’s t -test. How to cite this article : Jeong, M.-H. et al . Cdo suppresses canonical Wnt signalling via interaction with Lrp6 thereby promoting neuronal differentiation. Nat. Commun. 5:5455 doi: 10.1038/ncomms6455 (2014).